Polarization-controlled directional scattering for nanoscopic position sensing Controlling the propagation and coupling of light to sub-wavelength antennas is a crucial prerequisite for many nanoscale optical devices. Recently, the main focus of attention has been directed towards high-refractive-index materials such as silicon as an integral part of the antenna design. This development is motivated by the rich spectral properties of individual high-refractive-index nanoparticles. Here we take advantage of the interference of their magnetic and electric resonances to achieve strong lateral directionality. For controlled excitation of a spherical silicon nanoantenna, we use tightly focused radially polarized light. The resultant directional emission depends on the antenna’s position relative to the focus. This approach finds application as a novel position sensing technique, which might be implemented in modern nanometrology and super-resolution microscopy set-ups. We demonstrate in a proof-of-concept experiment that a lateral resolution in the Ångström regime can be achieved. Cylindrical vector beams are well-established tools in modern microscopy, ranging from scanning microscopy, where a reduced focal spot size can be achieved with a radially polarized beam [1] , [2] , [3] , [4] , to more sophisticated techniques such as stimulated-emission depletion [5] , [6] and multi-photon microscopy [7] . In addition, those polarization-tailored beams have also paved the way towards versatile applications in recent nanophotonic experiments by enabling selective excitation of nanoparticle eigenmodes [8] , [9] or controllable directional emission and waveguide-coupling of single plasmonic nanoantennas [10] . In this work, we combine several aspects of both research fields to present a novel approach towards high-precision position sensing, a discipline that is of paramount importance in modern nanometrology [11] , [12] , [13] , [14] , [15] , [16] , [17] , [18] , because of its special role in super-resolution microscopy [19] , [20] , [21] , [22] . Our all-optical technique for localization of a single nanoantenna is thereby based on encoding the position of the antenna in its laterally directional scattering pattern. For that purpose, we take advantage of the resonance properties of a high-refractive-index silicon nanoantenna featuring electric and magnetic resonances [23] , [24] , [25] , [26] . Excitation scheme It was shown that the simultaneous excitation of transverse electric and magnetic resonances of a high-refractive-index dielectric nanoparticle may yield enhanced or suppressed forward/backward scattering due to their interference [27] , [28] , [29] , [30] . However, by carefully structuring the excitation field three-dimensionally (3D) and thus also exciting longitudinal particle modes [9] , the scattering pattern can be tailored to achieve lateral directivity in the far field. For example, a tightly focused radially polarized beam features a promising 3D focal field with cylindrical symmetry [1] , [2] . 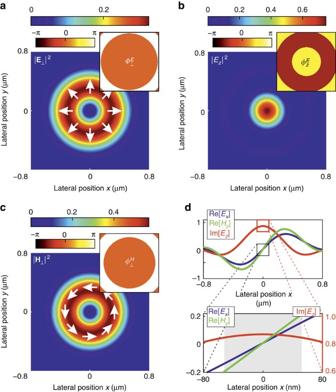Figure 1: Theoretical field intensity distributions and relative phases of a tightly focused radially polarized beam. The wavelengthλ=652 nm and experimental parameters are taken into account (see Methods section). (a) The transverse (radial) electric field intensity, (b) the longitudinal electric field intensityand (c) the transverse (azimuthal) magnetic fieldare all normalized to the maximum value of the total field intensity,(Gaussian units). The corresponding phase distributions,andare plotted as insets. (d) Cross-sections of the focal fields along thexaxis. Close to the centre (grey area in the lower image), the transverse field amplitudes Re[Ex] and Re[Hy] are linearly dependent on the position, while the longitudinal field Im[Ez] is approximately constant. Figure 1a–c shows its electric and magnetic field intensity distributions and the corresponding phases, calculated by vectorial diffraction theory [31] , [32] , while taking into account the experimental parameters. Apart from the transverse (in-plane) radially polarized electric field , a strong longitudinal component E z is formed, reaching its maximum amplitude on the optical axis. In contrast, the magnetic field is purely transverse and azimuthally polarized. In close vicinity to the optical axis, E z exhibits a phase delay of Δ φ z =± π /2 with respect to the transverse field components, and the electric and magnetic fields can be approximated by: Figure 1: Theoretical field intensity distributions and relative phases of a tightly focused radially polarized beam. The wavelength λ =652 nm and experimental parameters are taken into account (see Methods section). ( a ) The transverse (radial) electric field intensity , ( b ) the longitudinal electric field intensity and ( c ) the transverse (azimuthal) magnetic field are all normalized to the maximum value of the total field intensity, (Gaussian units). The corresponding phase distributions , and are plotted as insets. ( d ) Cross-sections of the focal fields along the x axis. Close to the centre (grey area in the lower image), the transverse field amplitudes Re[ E x ] and Re[ H y ] are linearly dependent on the position, while the longitudinal field Im[ E z ] is approximately constant. Full size image Here, , and are real valued amplitudes of the transverse electric, longitudinal electric and transverse magnetic field components, respectively, and ( x , y ) are Cartesian coordinates in the focal plane. Without loss of generality, the point in time is chosen such that the transverse field components E x , E y , H x and H y are real, and the longitudinal component E z is imaginary, owing to the aforementioned phase delay of π /2. For the chosen beam parameters (see Methods section), we estimate equations (1) and (2) to be valid within the region up to 50 nm away from the optical axis (see grey area in Fig. 1d ). In this limited range, the transverse electric and magnetic fields are linearly dependent on the coordinates x and y , while E z is assumed to be approximately constant. In order to adopt this linear position dependence of the transverse electromagnetic field for position sensing, a sub-wavelength antenna, capable of incorporating the local field in its far-field emission pattern, is required to localize the antenna unambiguously by its (directional) scattering pattern recorded in the far field. In the following, we discuss a silicon nanosphere (radius r =92 nm), whose spectrum in the visible range was experimentally investigated previously [9] , and we explain how its far-field emission pattern is governed by its position. 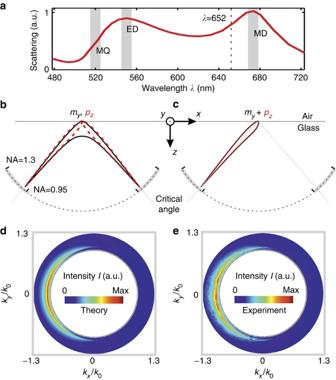Figure 2: Scattering of a silicon nanoantenna sitting on a dielectric interface. (a) Simulated scattering cross-section (linearly polarized Gaussian beam used for excitation) of a silicon sphere with radiusr=92 nm; only the forward scattering efficiency into the angular region within the NA∈[0.95, 1.3] is considered to match the experimental detection scheme (see grey arcs inb,c, and far-field patterns ind,e). In the visible range, the nanosphere supports magnetic dipole (λMD≈670 nm), electric dipole (λED≈550 nm) and magnetic quadrupole (λMQ≈520 nm) resonances. At the excitation wavelength ofλ=652 nm, the magnetic and electric dipole moments areπ/2 out of phase with respect to each other. (b) Emission of a longitudinal electric dipolepz(see dashed red line) and a transverse magnetic dipolemy(see black line) into the glass substrate. (c) In-phase far-field interference ofpzandmyresults in strong directivity. Comparison of (d) a calculated far-field pattern (interference ofpzandmy) and (e) a measured back-focal-plane image, retrieved at an antenna position on thexaxis 140 nm away from the centre of the beam. Tailored directional scattering Figure 2a shows the scattering cross-section of the antenna sitting on a glass substrate, simulated using the finite-difference time-domain method (similar to ref. 9 ). Here, only the forward scattering efficiency into the angular region within the numerical aperture (NA) ∈ [0.95, 1.3] is considered to match the experimental detection scheme described below (see also Fig. 2b–e ). In the visible spectral range, the silicon antenna supports the following three pronounced resonances: [9] the magnetic dipole ( λ MD ≈670 nm), the electric dipole ( λ ED ≈540 nm) and the magnetic quadrupole ( λ MQ ≈515 nm). For wavelengths above 600 nm, the weak contribution of the magnetic quadrupole can be completely neglected [9] , and the antenna can be approximated by a point-like dipole (electric and magnetic). Assuming that the dipole moments are proportional to the respective local field vectors, p ∝ E and m ∝ H , we yield the position-dependent dipole moments and . The aim of our experimental concept is to achieve highly position-sensitive far-field directivity caused by the interference of the, in first approximation, constant z -oriented electric dipole p z and the position-dependent transverse components of the magnetic dipoles m x and m y . The influence of the transverse electric dipole components p x and p y will be proven to be negligible later on. Figure 2: Scattering of a silicon nanoantenna sitting on a dielectric interface. ( a ) Simulated scattering cross-section (linearly polarized Gaussian beam used for excitation) of a silicon sphere with radius r =92 nm; only the forward scattering efficiency into the angular region within the NA ∈ [0.95, 1.3] is considered to match the experimental detection scheme (see grey arcs in b , c , and far-field patterns in d , e ). In the visible range, the nanosphere supports magnetic dipole ( λ MD ≈670 nm), electric dipole ( λ ED ≈550 nm) and magnetic quadrupole ( λ MQ ≈520 nm) resonances. At the excitation wavelength of λ =652 nm, the magnetic and electric dipole moments are π /2 out of phase with respect to each other. ( b ) Emission of a longitudinal electric dipole p z (see dashed red line) and a transverse magnetic dipole m y (see black line) into the glass substrate. ( c ) In-phase far-field interference of p z and m y results in strong directivity. Comparison of ( d ) a calculated far-field pattern (interference of p z and m y ) and ( e ) a measured back-focal-plane image, retrieved at an antenna position on the x axis 140 nm away from the centre of the beam. Full size image In Fig. 2b , the far-field intensities of a z -oriented electric dipole (see dashed red line) and a y -oriented magnetic dipole (see black line) emitted into the glass substrate are depicted. Here, we consider the electric and magnetic dipole moments to exhibit the same strength. If the dipole moments are in phase, the interference of both far fields yields a remarkably strong lateral directivity ( Fig. 2c ). Figure 2d shows the corresponding calculated k -spectrum in the experimentally accessible region within NA ∈ [0.95, 1.3]. At this point, the relative phase between the longitudinal and the transverse field components (Δ φ z =± π /2, see insets in Fig. 1 ) of the excitation beam needs to be considered. If the electric and magnetic dipoles oscillate π /2 out of phase, no directivity would be observed in the far field because their symmetric far-field intensity distributions add up. Hence, an additional phase of π /2 is required to compensate for Δ φ z . Since the relative phase between a dipole moment and its respective excitation field (Δ φ MD for the magnetic, Δ φ ED for the electric field) depends on the wavelength, we can compensate for Δ φ z by carefully choosing the wavelength of the incoming light with respect to the spectral positions of the electric and magnetic dipole resonances. From simulation, we retrieve the relative phase between the electric and magnetic dipole moment to be Δ φ =Δ φ MD −Δ φ ED = π /2 for a wavelength of λ =652 nm ( Supplementary Fig. 1 and Supplementary Note 1 ). Using this wavelength for excitation, we expect to achieve strongly directional scattering at antenna positions where the longitudinal electric and transverse magnetic fields overlap. For experimental verification, a measured far-field image is plotted in Fig. 2e . The image was retrieved by placing the antenna on the x axis ∼ 140 nm away from the centre of the beam in the focal plane, effectively obtaining longitudinal electric and transverse magnetic dipole moments of equal strength. The strong directivity proves that the compensation of the relative phase has been successful, and the very good overlap of 94% with the theoretical pattern suggests that, in first-order approximation, the transverse electric dipole moments, not taken into account here, can indeed be neglected (details can be found in Supplementary Fig. 2 and Supplementary Note 2 ). In short, we optimized the polarization distribution and the wavelength of our excitation beam to achieve strongly directional emission depending on the position of a single silicon nanoantenna relative to the beam’s optical axis. The underlying principle causing the directivity is the simultaneous and in-phase excitation of a longitudinal electric and a transverse magnetic dipole moment. Experimental implementation and calibration A sketch of the experimental set-up is depicted in Fig. 3a (for more details see ref. 33 ). The collimated incoming radially polarized beam ( λ =652 nm) was tightly focused by a microscope objective with an NA of 0.9 onto the silicon nanosphere sitting on a glass substrate (see electron micrograph in Fig. 3a ), which was positioned precisely within the focal plane by a 3D piezo-stage. A second microscope objective (oil-immersion type, NA=1.3) below the substrate collected both the transmitted beam and the forward scattered light. Imaging the back-focal plane of the second microscope objective onto a CCD camera enabled acquisition of the intensity distribution emitted into the far field and grants access to the angular spectrum of the scattered field (see examples in Figs 2e and 3b,c ). Similar to ref. 10 , only the region of NA ∈ [0.95, 1.3] was considered, where the scattered light can be detected without interfering with the transmitted beam. 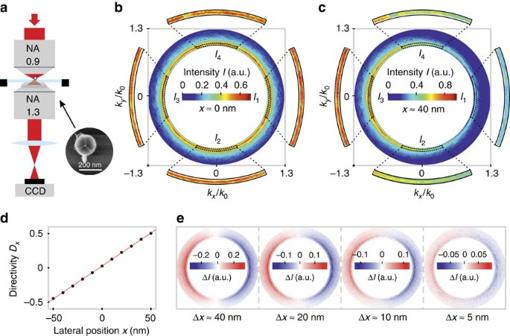Figure 3: Set-up and experimental results. (a) A radially polarized collimated beam is tightly focused by a microscope objective (NA=0.9) onto a sub-wavelength silicon antenna sitting on a glass substrate (see inset). The light emitted into the angular regime with NA∈[0.95, 1.3] is collected by an oil-immersion type microscope objective (NA=1.3). The back-focal plane is imaged onto a CCD camera. (b) Acquired far-field intensity distributionI(kx,ky) for the antenna placed on the optical axis and (c) for the antenna displaced laterally byx≈40 nm (off-axis). The dashed black lines and the magnified insets indicate four regions with averaged intensitiesI1,I2,I3andI4. (d) Directivity parameterDxversus the antenna’s position along thexaxis; the slope of the curve (0.01 nm−1) defines the sensitivity of the measurement to the antenna displacement. (e) Far-field intensity difference images for four antenna positions along thexaxis (left to right: Δx≈40, 20, 10 and 5 nm away from the optical axis). The left image corresponds to the intensity difference ΔI(kx,ky) betweenb,c. Figure 3: Set-up and experimental results. ( a ) A radially polarized collimated beam is tightly focused by a microscope objective (NA=0.9) onto a sub-wavelength silicon antenna sitting on a glass substrate (see inset). The light emitted into the angular regime with NA ∈ [0.95, 1.3] is collected by an oil-immersion type microscope objective (NA=1.3). The back-focal plane is imaged onto a CCD camera. ( b ) Acquired far-field intensity distribution I ( k x , k y ) for the antenna placed on the optical axis and ( c ) for the antenna displaced laterally by x ≈40 nm (off-axis). The dashed black lines and the magnified insets indicate four regions with averaged intensities I 1 , I 2 , I 3 and I 4 . ( d ) Directivity parameter D x versus the antenna’s position along the x axis; the slope of the curve (0.01 nm −1 ) defines the sensitivity of the measurement to the antenna displacement. ( e ) Far-field intensity difference images for four antenna positions along the x axis (left to right: Δ x ≈40, 20, 10 and 5 nm away from the optical axis). The left image corresponds to the intensity difference Δ I ( k x , k y ) between b , c . Full size image To retrieve the position of the antenna from the back-focal plane images, we averaged the measured intensity over four small regions in k -space (black dotted lines in Fig. 3b,c ) [34] , resulting in four averaged intensity values I 1 , I 2 , I 3 and I 4 . The size and position of these four regions was chosen to include only the strongest change of the far-field intensity for an antenna shift along the x or y axis. The normalized intensity differences and , with , represent directivity parameters, which are linear functions of the antenna position ( Supplementary Note 3 ). In order to compensate for experimental imperfections such as beam aberrations or deviations from the ideal antenna shape, the measurement approach requires initial calibration, for which we placed the antenna centrally in the focus. At this position, the far-field distribution of the scattered light is expected to be cylindrically symmetric, since only a longitudinal electric dipole moment can be excited ( Fig. 3b ) [9] , [10] . From this reference point, the antenna was scanned across the focal plane (100 × 100 nm), with a step-size of 10 nm. For each position, an image of the back-focal plane was acquired and the corresponding values of D x and D y were determined. The whole procedure was repeated 40 times and the measured directivity parameters were averaged in order to decrease the influence of the instability of our set-up (position uncertainty of ±5 nm). Thereupon, linear equations were fitted to the averaged directivity parameters D x ( x , y ) and D y ( x , y ) (see equation (8) in the Methods section), which allow for retrieving the antenna position from individual back-focal plane images. As an example, Fig. 3d shows the averaged directivity parameter D x plotted against the x coordinate and the corresponding linear fit. Lateral resolution In order to demonstrate the accuracy in the measurement of the antenna position, which can be achieved with a single camera shot, far-field images for different antenna positions are analysed. To this end, we normalize the intensity maps recorded in each back-focal plane to the intensity and calculate the difference to a reference image, which corresponds to the antenna sitting on the optical axis ( Fig. 3b ). For the demonstration of this inherently 2D localization technique, we show results for x displacements only. In Fig. 3e , we depict four post-selected difference images for the antenna being placed on the x axis, for which our calibration measurement indicated relative positions of Δ x ≈40, 20, 10 and 5 nm (Δ y ≈0 nm). For a relatively large displacement of Δ x ≈40 nm, the difference image corresponding to the difference between Fig. 3b,c yields a very good signal-to-noise ratio. Even for a small displacement of only Δ x ≈5 nm, the difference image reveals predominately negative values on the left side ( k x <0) and positive values on the right side ( k x >0). However, the signal-to-noise ratio decreases with shorter distances Δ x . The theoretical limit of our resolution is determined by the derivatives (slopes) of D x ( x , y ) and D y ( x , y ), the intensity noise of an individual camera pixel, and the actual number of pixels in each integration region. Our calculations yield that a position uncertainty below 2 Å could be achieved. More details and an actual experimental example can be found in Supplementary Fig. 3 and Supplementary Note 4 . However, a direct proof of this accuracy would require a highly stabilized set-up including a piezo-stage with Ångström precision. In summary, we experimentally demonstrated that the simultaneous and phase-adapted excitation of longitudinal electric and transverse magnetic dipole modes of a high-refractive-index nanosphere yields extraordinarily strong directionality. Especially the spectral tuning of the relative phase between both dipole modes in combination with the appropriate choice of a 3D focal field pattern enabled highly position-sensitive transverse scattering directionality. We utilized the approach as a novel technique for single-shot lateral position sensing, achieving localization accuracies down to a few Ångström, which is comparable to other state-of-the-art localization methods presented in literature [12] , [13] , [18] . Our technique could be applied for the stabilization of samples, for instance, in super-resolution microscopy. Furthermore, since the directionality is also present in the super-critical regime (NA>1), evanescent coupling to waveguide modes will allow for on-chip detection of the directional scattering and, hence, of the lateral position of the sample. Finally, future studies might demonstrate that antenna design and size, as well as the excitation field can be optimized to achieve an even stronger dependence of the directionality on the particle position, which would allow for sub-Ångström localization accuracies. Experimental set-up A tunable light source (NKT Photonics SuperK Extreme & SpectraK Dual) emits a linearly polarized Gaussian beam at a wavelength of 652 nm, which is converted into a radially polarized beam by a liquid-crystal polarization converter (q-plate) [35] , [36] . The beam with radius w 0 =1.26 mm is then guided into a microscope objective with NA=0.9 and an entrance aperture radius of 1.8 mm (Leica HCX PL FLUOTAR 100 × /0.90 POL 0/D). A single spherical silicon nanoparticle with radius r =92 nm on a glass substrate is scanned through the focal plane by a high-precision 3D piezo-stage (PI P-527), and the transmitted light is collected with an oil-immersion objective with NA=1.3 (Leica HCX PL FLUOTAR 100 × /1.30 OIL). The angular intensity distribution of the transmitted light is detected by imaging the back-focal plane of the oil-immersion objective onto a CCD camera (The Imaging Source DMK 23U618). The four solid angles corresponding to I 1 , I 2 , I 3 and I 4 (see dashed lines in Fig. 3b,c ) are defined by an azimuthal angular range of ΔΦ=45° and by NA ∈ [0.98, 1.02]. Calculation of the far-field distribution We make use of the cylindrical symmetry of the beam and, without loss of generality, only consider antenna positions along the x axis. Therefore, only the longitudinal electric ( p z ) and transverse magnetic ( m y ) dipole moments need to be considered. The transverse electric (s-polarized) and transverse magnetic (p-polarized) far-field distributions emitted into the dielectric substrate (refractive index n =1.5) are expressed in ref. 32 . with the Fresnel coefficients for transmission t p and t s , the wavenumber in vacuum k 0 =2 π / λ , the transverse component of the k -vector and the vacuum speed of light c 0 . Comparison between theoretical and experimental far-field patterns enables estimating the distance between the effective point-like dipole and the interface, d =70 nm. The emission patterns in Fig. 2b,c are calculated using equations (3)–(6), whereby we considered a similar strength for both dipole moments p z = m y / c 0 to achieve maximum directivity. Taking into account the aplanatic microscope objective, an additional energy conservation factor proportional to is introduced for Fig. 2d (ref. 32 ). Calibration measurement The directivity parameters D x and D y are linear functions of the lateral antenna position x and y , respectively. Thus, we fit a system of two linear equations to the averaged calibration measurement data, resulting in Ideally, the matrix has non-zero values on its diagonal only. The small off-diagonal elements indicate a minor rotation of the coordinate system and, in addition, not entirely orthogonal directivity parameters D x and D y . The rotation of the coordinates might stem from a misalignment of our camera with respect to the coordinate frame of the piezo-stage, while the non-orthogonal basis can be related to aberrations of the beam and asymmetries of the antenna (see electron micrograph in Fig. 3a ). The derivatives (slopes) of D x and D y define the sensitivity of the directivity to a displacement of the antenna. At the rim of the region of linearity, 50 nm away from the centre, we already achieve a directivity D x =48% ( D y =52%) if the antenna is shifted in x direction ( y direction). Post-selection of difference images The instability of our experimental set-up causes an uncertainty of ±5 nm regarding the position of the particle relative to the beam. For this reason, we took 40 individual images for each position set by the piezo-stage (Δ x ≈40, 20, 10 and 5 nm), and then post-selected the far-field images of which the directivity parameters D x and D y best-represented the position set by the piezo-stage according to the calibration measurement (equation (8)). Finally, we calculated the difference images depicted in Fig. 3e . How to cite this article: Neugebauer, M. et al . Polarization-controlled directional scattering for nanoscopic position sensing. Nat. Commun. 7:11286 doi: 10.1038/ncomms11286 (2016).